Meta-analysis of genome-wide association studies identifies novel loci that influence cupping and the glaucomatous process Glaucoma is characterized by irreversible optic nerve degeneration and is the most frequent cause of irreversible blindness worldwide. Here, the International Glaucoma Genetics Consortium conducts a meta-analysis of genome-wide association studies of vertical cup-disc ratio (VCDR), an important disease-related optic nerve parameter. In 21,094 individuals of European ancestry and 6,784 individuals of Asian ancestry, we identify 10 new loci associated with variation in VCDR. In a separate risk-score analysis of five case-control studies, Caucasians in the highest quintile have a 2.5-fold increased risk of primary open-angle glaucoma as compared with those in the lowest quintile. This study has more than doubled the known loci associated with optic disc cupping and will allow greater understanding of mechanisms involved in this common blinding condition. Optic nerve degeneration caused by glaucoma is the most common cause of irreversible blindness worldwide [1] . Glaucomatous optic neuropathy is recognized by changes in the morphology of the optic nerve head, or optic disc, caused by loss of retinal ganglion cells and thinning of the retinal nerve fibre layer. In glaucoma, the nerve fibre layer typically thins in the superior and inferior regions of the nerve creating a vertically elongated depression (the cup). The ratio of the cup to the overall nerve size (the disc), called the vertical cup-disc ratio (VCDR), is a key factor in the clinical assessment and follow-up of patients with glaucoma. VCDR has been shown to be heritable with h 2 scores ranging between 0.48 and 0.66 [2] , [3] , [4] , [5] , [6] , [7] . At least seven loci have been associated with VCDR in previous genome-wide association studies (GWAS) and three of these were subsequently implicated in primary open-angle glaucoma (POAG) [8] , [9] , [10] , [11] . So far, the explained variance of open-angle glaucoma by age, sex, intraocular pressure and established POAG genes is still small (4–6%) [12] . As with other complex diseases, large sample sizes are needed to ensure sufficient power to fully define the underlying genetic architecture. Here, we report the largest genome-wide meta-analysis for VCDR, with data from 14 studies from Europe, the United States, Australia and Asia, as part of the International Glaucoma Genetics Consortium. The aim of the study is to identify loci associated with VCDR, and to determine whether these variants are also associated with glaucoma. We perform the meta-analysis in four stages. In the first stage, we meta-analyse summary data from 10 populations of European ancestry comprising 21,094 individuals. In the second stage, we test the cross-ancestry transferability of the statistically genome-wide-significant associations from the first stage in 6,784 individuals from four Asian cohorts. In the third stage, we examine whether the associations are independent of disc area and/or spherical equivalent. We also combine the genome-wide-significant effects into a genetic risk score and associate this score with the POAG risk in five populations. Finally, we perform gene-based tests and pathway analysis. We find 10 new loci associated with VCDR, which together increase the risk on POAG 2.5 times. Our findings will help us to unravel the pathogenesis of glaucoma. Meta-analysis of GWAS In stage 1, we analysed ~2.5 million HapMap stage 2 single-nucleotide polymorphisms (SNPs)—either directly genotyped or imputed in 21,094 subjects of European ancestry ( Supplementary Fig. 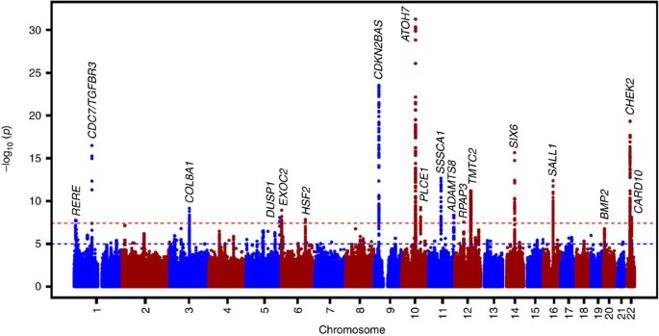Figure 1: Manhattan plot of the GWAS meta-analysis for vertical cup-disc ratio in the combined analysis (n=27,878). The plot shows −log10-transformedPvalues for all SNPs (z-statistic). The red-dotted horizontal line represents the genome-wide significance threshold ofP<5.0 × 10−8; the blue-dotted line indicatesPvalue of 1 × 10−5. 1 ; Supplementary Table 1 ; Supplementary Methods ). The inflation factors ( λ ) varied between 0.98 and 1.12, implying adequate within-study control of population substructure ( Supplementary Table 2 ; Supplementary Figs 2 and 3 ). The overall λ was 1.05. This analysis yielded 440 genome-wide-significant SNPs ( P <5.0 × 10 −8 ) located across 15 chromosomal regions ( Table 1 ; Supplementary Fig. 4a ). In stage 2, we investigated the SNP with the strongest association at each region in the Asian populations and found that eight were nominally significant ( P <0.05) with an effect in the same direction and generally the same order of magnitude ( Table 1 ; Supplementary Fig. 4b ). Five of the seven loci that did not reach nominal significance in those of Asian descent had a similar effect in the same direction. Supplementary Table 3 shows the most significant SNPs in Asians within 100,000 base pairs from the most significant associated SNP in Europeans. Meta-analysis of only the Asian populations did not result in new genome-wide-significant findings. The combined analysis of the European and Asian populations resulted in three additional genome-wide-significant associations on chromosomes 1, 6 and 22 ( Table 1 ; Fig. 1 ). The level of heterogeneity across the samples are shown in Table 1 . Of the 18 genome-wide-significant loci, 10 are novel for the VCDR outcome ( COL8A1 , DUSP1 , EXOC2 , PLCE1 , ADAMTS8 , RPAP3 , SALL1 , BMP2 , HSF2 and CARD10 ) ( Supplementary Fig. 5 ). There were no significant differences in terms of allele frequencies across the different cohorts ( Supplementary Table 4 ). The effect estimates from the participating cohorts appear not to be influenced by main demographic characteristics, such as mean age and sex ratio ( Supplementary Fig. 6 ). Table 1 Summary of the results of the meta-analyses of genome-wide association studies. Full size table Figure 1: Manhattan plot of the GWAS meta-analysis for vertical cup-disc ratio in the combined analysis ( n =27,878). The plot shows −log 10 -transformed P values for all SNPs ( z -statistic). The red-dotted horizontal line represents the genome-wide significance threshold of P <5.0 × 10 −8 ; the blue-dotted line indicates P value of 1 × 10 −5 . Full size image Adjustment for disc area and spherical equivalent Four of the 18 genome-wide-significant loci have been previously associated with optic disc area ( CDC7/TGFBR3 , ATOH7 , SALL1 and CARD10 ) [10] , [13] . Because the size of the optic nerve varies between individuals and is correlated to the VCDR [14] , we adjusted the association to VCDR for optic nerve (disc) area. This resulted in a reduced effect size and significance ( P =3.48 × 10 −11 to P =9.00 × 10 −3 ) at the CDC7–TGFBR3 locus, suggesting the VCDR association at this locus is explained primarily by its known association with disc area ( Supplementary Table 5a–c ). A similar reduction in effect was seen for ATOH7 . However, for this locus there remains a significant disc-area-independent effect ( P =7.28 × 10 −9 ). There was no change in association significance for any of the 10 new loci reported here, suggesting they do not act primarily on disc area. It is of interest that two genes ( SIX6 and BMP2 ) overlap with those implicated in myopia [15] , an important risk factor for POAG [16] . The correlation between VCDR and spherical equivalent is low ( Supplementary Table 6 ), and adjusting for spherical equivalent did not lead to any major changes in the effects for these or other loci in European populations ( Supplementary Table 7a ), suggesting a joint genetic aetiology for POAG and myopia. In Asian cohorts, the direction of effect on VCDR at the chromosome 11 locus ( MIR612-SSSCA1 region) was not consistent with the European populations ( Supplementary Table 7b ). However, after adjusting for spherical equivalent the direction of effect on VCDR was similar to both populations. At the BMP2 myopia locus, we observed a large difference in allele frequency between those of European and Asian ancestry ( Table 1 ), which may explain the difference in effect direction. Risk for POAG The 18 loci, together with age and sex, explain 5.1–5.9% of the VCDR phenotypic variability in Europeans (measured in the Rotterdam Study I, II and III), of which 1.6–1.8% is explained by the new loci. The phenotypic variability explained by all common SNPs is 41–53% in these cohorts, which is in line with the heritability estimates from family-based studies. In addition to confirming the previously published CDKN2BAS and SIX1/6 POAG risk loci, we found nominally significant ( P <0.05) associations with POAG for six newly identified genetic variants ( P =8.1 × 10 −5 from binomial test for chance of seeing six or more such nominally significant associations in 16 tests) ( Supplementary Table 8 ), with odds ratios varying between 0.73 and 1.20. In the combined case-control studies, we found that the sum of all effects of these genes increased the risk of POAG 2.5-fold ( Supplementary Table 9 ) for those in the highest quintile compared with those in the lowest quintile. Gene-based test To identify new loci not previously found through individual SNP-based tests, we performed gene-based tests using VEGAS software [17] . Because of the smaller number of tests (17,872 genes tested), our gene-based significance threshold is P gene-based <0.05/17,872=2.80 × 10 −6 . In addition to the SNPs identified as significant ( P <5 × 10 −8 ) in a SNP-based test, we also found two new genes significantly associated with VCDR using the VEGAS gene-based test ( Supplementary Table 10 ). These were REEP5 ( P =7.48 × 10 −7 ) and PITPNB ( P =4.89 × 10 −7 ). PITPNB is ~800 kb from another gene with a significant SNP association ( CHEK2 , rs1547014) ( Supplementary Fig. 7 ). Although the association signal centred over CHEK2 extends a long distance towards PITPNB , a separate association peak over PITPNB can be observed, which is unrelated (no linkage disequilibrium (LD)) to the CHEK2 peak. The results we obtained using the specified definition of the gene unit were substantially the same when alternative cutoff points from the transcription initiation and end sites were used ( Supplementary Table 11 ). The REEP5 gene showed no association with POAG ( Supplementary Table 12 ). The PITPNB gene showed evidence for association with POAG in Australian & New Zealand Registry of Advanced Glaucoma (ANZRAG) ( P =0.03) in the gene-based test, with a best single SNP P value of 0.003, but this was not confirmed in two other studies. Pathway analysis To test whether gene-based statistics identified were enriched in 4,628 pre-specified Gene Ontology pathways, we performed pathway analysis using Pathway-VEGAS [18] . We used a pathway-wide significance threshold to be 1.08 × 10 −5 (0.05/4,628). The only pathway exceeding the pathway-wide significance level was ‘negative regulation of cyclin-dependent protein kinase activity’ ( Supplementary Table 13 ). The second top-pathway ‘negative regulation of epithelial cell proliferation’ is related to the top pathway, both suggesting retardation of cell growth. The ‘negative regulation of cyclin-dependent protein kinase activity’ finding was driven not only by the result at the CDKN2A locus but also by the result at APC , a gene close to REEP5 . Regulatory elements and expression data Six of the 18 most associated SNPs are located in DNase I hypersensitivity sites ( Supplementary Table 14 ). The retinal pigment epithelium has the highest signal of all 125 available cell lines in one of these DNase I hypersensitivity sites. Thus, these results are suggesting that some of the SNPs may have their effect on VCDR by altering regulatory functions. We investigated the expression of the genes implicated in VCDR by these analyses in human ocular gene expression databases or the published literature. Most of these genes are expressed in eye tissues, including the optic nerve ( Supplementary Tables 15 and 16 ). This study reports 10 novel loci associated with VCDR, with an additional two loci identified using gene-based testing. Pathway analysis suggests retardation of cell growth as a major biological mechanism. The results for the most associated pathways ‘negative regulation of cyclin-dependent protein kinase activity’ and ‘negative regulation of epithelial cell proliferation’ are primarily driven by the CDKN2A and CDKN2B genes, respectively, but in both pathways the gene-based result at APC ( P =7.20 × 10 −5 in Caucasians and P =8.80 × 10 −3 in Asians) also contributes to the pathway result. The APC gene has previously been reported to be a critical gene regulating retinal pigment epithelium proliferation and development [19] . These results add to our earlier findings on the role of growth and the transforming growth factor beta (TGFB) pathways in VCDR [10] . Various new genes fall into these pathways. The protein encoded by the BMP2 (bone morphogenetic protein 2) gene on chromosome 20 belongs to the TGFB super-family. Two other new genes regulate apoptosis: RPAP3 (RNA polymerase II-associated protein 3) on chromosome 12 [20] and CARD10 , a gene that was previously found to be associated with disc area [13] . Another new VCDR association previously associated with disc area is SALL1 [10] . This gene is implicated in ocular development. Our findings offer new insights in the aetiology of optic nerve degeneration. COL8A1 (collagen, type VIII, alpha 1) is part of a collagen pathway recently implicated in corneal thickness [18] , an ocular trait also associated with glaucoma risk. Missense mutations in COL8A2 (collagen, type VIII, alpha2) were found in POAG patients with a very thin central corneal thickness (CCT) [21] . The collagen SNP (rs2623325) was not significantly associated with CCT (in Caucasians: β =−0.044, P =0.19; in Asians: β =0.007, P =0.89) or intraocular pressure (in Caucasians and Asians combined: β =−0.02, P =0.73) in largely the same cohorts [18] , [22] , suggesting that the collagen involvement in VCDR is not due to the influence by CCT or intraocular pressure. We also found several genes involved in cellular stress response. DUSP1 (dual specificity phosphatase 1) is the nearest gene to the most strongly associated SNP on chromosome 5. This gene, inducible by oxidative stress and heat shock, may play a role in environmental stress response [23] , and may also participate in the negative regulation of cellular proliferation. HSF2 (heat shock transcription factor 2), one of the genes at the chromosome 6 locus, also is part of the cellular stress response pathway. Deficiency of this factor causes various central nervous system defects in mice [24] , [25] . Another pathway emerging in this study is that of exocytosis. The SNP on the other chromosome 6 locus is located in EXOC2 (exocyst complex component 2). The encoded protein is one of the eight proteins of the exocyst complex [26] . This multi-protein complex is important for directing exocytic vesicles to the plasma membrane, a mechanism that also has been implicated in neuronal degeneration in the brain [27] . Lipid metabolism emerges as another pathway. The gene on chromosome 10, PLCE1 (phospholipase C, epsilon 1), belongs to the phospholipase C family, which plays a role in the generation of second messengers [28] . Various processes affecting cell growth, differentiation and gene expression are regulated by these second messengers. From a clinical perspective, the findings on ADAMTS8 are of interest. ADAMTS enzymes have different functions, including the formation and turnover of the extracellular matrix [29] . Strikingly, a variant in ADAMTS10 has been linked to a form of glaucoma in dogs [30] , [31] . In summary, we have now identified 10 novel loci associated with cupping of the optic nerve, a key determinant of glaucoma. Together, these genetic risk variants increased the risk of POAG in case-control validation studies. Pathway analysis implicated negative regulation of cell growth and cellular response to environmental stress as key pathological pathways in glaucoma, and that novel therapies targeting these pathways may be neuro-protective in glaucoma. Study design We performed a meta-analysis on directly genotyped and imputed SNPs from individuals of European ancestry in 10 studies, with a total of 21,094 individuals. Subsequently, we evaluated significantly associated SNPs in 6,784 subjects of Asian origin including four different studies and performed a meta-analysis on all studies combined. Subjects and phenotyping All studies included in this meta-analysis are part of the International Glaucoma Genetics Consortium. The ophthalmological examination of each study included an assessment of the optic nerve head to measure the VCDR ( Supplementary Table 17a ). Unreliable optic nerve data were excluded. The meta-analysis of stage 1 was based on 10 studies of European ancestry: Brisbane Adolescent Twin Study, Blue Mountains Eye Study, Erasmus Rucphen Family Study, Gutenberg Health Study (GHS I/GHS II), Glaucoma Genes and Environment (controls only), National Eye Institute Glaucoma Human Genetics Collaboration (NEIGHBOR; controls only), Raine Study, Rotterdam Study (RS-I/RS-II/RS-III), Twins Eye Study in Tasmania and TwinsUK. Stage 2 comprised four Asian studies: Beijing Eye Study, Singapore Chinese Eye Study, Singapore Malay Eye Study and Singapore Indian Eye Study. For each SNP with the strongest association at each locus the association with POAG was tested in five case-control studies: ANZRAG, deCODE, Massachusetts Eye and Ear Infirmary, NEIGHBOR and Southampton. Information on general methods, demographics, phenotyping and genotyping methods of the study cohorts can be found in Supplementary Tables 1 and 17 and the Supplementary Note . All studies were performed with the approval of their local medical ethics committee, and written informed consent was obtained from all participants in accordance with the Declaration of Helsinki. Genotyping and imputation Information on genotyping in each cohort and the particular platforms used to perform genotyping can be found in more detail in Supplementary Table 17b . To produce consistent data sets and enable a meta-analysis of studies across different genotyping platforms, the studies performed genomic imputation on available HapMap Phase 2 genotypes with MACH [32] or IMPUTE [33] , using the appropriate ancestry groups as templates. Each study applied stringent quality control procedures before imputation, including minor allele frequency cutoffs, Hardy–Weinberg equilibrium, genotypic success rate, mendelian inconsistencies, exclusion of individuals with >5% shared ancestry (exception made for family-based cohorts in which due adjustment for family relationship was made) and removal of all individuals whose ancestry as determined through genetic analysis did not match the prevailing ancestry group of the corresponding cohort ( Supplementary Note ). SNPs with low imputation quality were filtered using metrics specific to the imputation method and thresholds used in previous GWAS analyses. For each cohort, only SNPs with imputation quality scores >0.6 (proper-info of IMPUTE) or R2>0.6 (MACH) were included into the meta-analysis. Statistical analysis In subjects drawn from their respective populations in which the prevalence of glaucomatous changes is relatively low, the correlation between left and right eye is high [34] . Therefore, we used the mean VCDR of both eyes. In cases of missing or unreliable data for one eye, data of the other eye was taken. Each individual study did a linear regression model between the VCDR and the SNPs under the assumption of an additive model for the effect of the risk allele. Analyses were adjusted for age, sex and the first two principal components (for population-based studies) or family structure (for family-based studies). Secondary analyses were done with adjustments for disc area or spherical equivalent. In the Rotterdam Studies, we calculated the phenotypic variability explained by the new loci, and explained by all common SNPs using the ‘Genome-wide Complex Trait Analysis’ tool [35] , [36] . We performed an inverse variance weighted fixed-effect meta-analysis. This was performed with METAL software [37] . P values for the association results were calculated by using the z -statistic. P values for heterogeneity were calculated by using the Cochran’s Q -test for heterogeneity. In addition to this, I 2 values were calculated to assess heterogeneity [38] . F st values were calculated to assess the genetic variation due to subdivision of populations. All study effect estimates were corrected using genomic control and were oriented to the positive strand of the NCBI Build 36 reference sequence of the human genome, which was the genomic build on which most available genotyping platforms were based. Coordinates and further annotations for the SNPs were converted into Build 37, the most recent version of the available builds at the time of this study. In stage 1, a P value <5.0 × 10 −8 (the genome-wide threshold of association) was considered significant. In stage 2, a P value <0.05 was considered significant. Manhattan, regional and forest plots were made using R [39] , LocusZoom [40] and Stata/SE 12.0 (StataCorp LP, College Station, TX, USA). Risk-score models In five case-control studies, a weighted genetic risk score per individual was calculated. Standardized regression coefficients were used as weighting factor. The weighted risk scores were divided into quintiles. Odds ratios were calculated for each quintile, using the first quintile as a reference. Gene-based test using VEGAS There are different gene-based tests of which VEGAS is one of the most powerful tests [41] . We therefore performed gene-based testing using VEGAS software [17] , which combines the test statistics of all SNPs present within and 50 kb upstream/downstream of each gene. LD between the markers is accounted for through simulations from the multivariate normal distribution, based on estimates of LD from reference populations. Since Asian and European ancestry populations show different LD patterns, we performed separate gene-based tests for each population. Hapmap 2 CEU population was used as a reference to calculate LD for European ancestry data, whereas Hapmap 2 JPT and CHB combined population was used as a reference for Asian ancestry data. After calculation of gene-based test statistics for Asian and European ancestry populations separately, meta-analysis was conducted using Fisher’s method for combining P values. VEGAS was applied to the summary data from the full VCDR analysis (as in Table 1 ) and to three of the POAG data sets; ANZRAG, Massachusetts Eye and Ear Infirmary glaucoma clinic and Glaucoma Genes and Environment ( Supplementary Note ). Pathway-analysis using pathway-VEGAS Pre-specified pathways from the Gene Ontology database with size ranging in 5–500 genes were used to perform pathway analysis. Pathway-VEGAS combines VEGAS gene-based test statistics based on pre-specified biological pathways [18] . Pathway P values were computed by summing χ 2 -test statistics derived from VEGAS P values. Empirical ‘VEGAS-pathway’ P values for each pathway were computed by comparing the real-data-summed χ 2 -test statistics with 500,000 simulations where the relevant number (as per size of pathway) of randomly drawn χ 2 -test statistics was summed. To ensure clusters of genes did not adversely affect results, within each pathway, gene sets were pruned such that each gene was >500 kb from all other genes in the pathway. Where required, all but one of the clustered genes was dropped at random when genes were clustered. Pathway-VEGAS was performed separately for European and Asian ancestry data sets. Meta-analysis was conducted using Fisher’s method for combining P values. Regulatory functions We used the ENCyclopedia Of DNA Elements [42] data in the UCSC Genome Browser [43] to look at DNase I hypersensitivity sites and other functional elements. Gene expression in human eye tissue We examined the expression of genes that reached significance in the individual SNP-based test or gene-based test. We used published literature or human ocular gene expression databases ( Supplementary Tables 15 and 16 ). How to cite this article: Springelkamp, H. et al . Meta-analysis of genome-wide association studies identifies novel loci that influence cupping and the glaucomatous process. Nat. Commun. 5:4883 doi: 10.1038/ncomms5883 (2014).